Oxygen induced promotion of electrochemical reduction of CO2via co-electrolysis 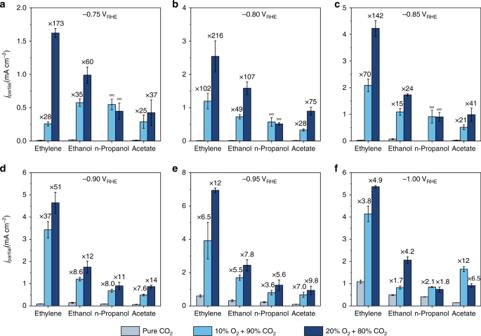Fig. 1: Comparison of C2+product formations. The partial current densities of C2+products measured at 100% CO2, 10% O2+ 90% CO2, and 20% O2+ 80% CO2are compared at different potentials ofa−0.75 VRHE,b−0.80 VRHE,c−0.85 VRHE,d−0.90 VRHE,e−0.95 VRHE, andf−1.0 VRHE. The numbers stand for the enhancement relative to the rates at pure CO2. The error bars represent the standard deviation from at least three independent measurements. 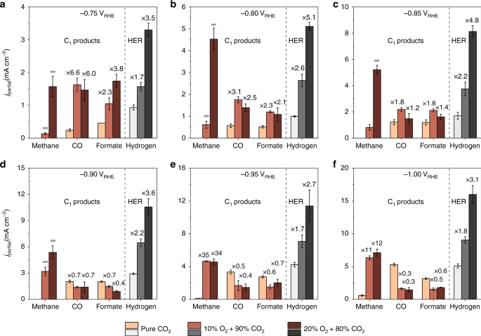Fig. 2: Comparison of C1product and H2formations. The partial current densities of C1products and H2measured at 100% CO2, 10% O2+ 90% CO2, and 20% O2+ 80% CO2are compared at different potentials ofa−0.75 VRHE,b−0.80 VRHE,c−0.85 VRHE,d−0.90 VRHE,e−0.95 VRHE, andf−1.0 VRHE. The numbers stand for the enhancement relative to the rates at pure CO2. The error bars represent the standard deviation from at least three independent measurements. Harnessing renewable electricity to drive the electrochemical reduction of CO 2 is being intensely studied for sustainable fuel production and as a means for energy storage. Copper is the only monometallic electrocatalyst capable of converting CO 2 to value-added products, e.g., hydrocarbons and oxygenates, but suffers from poor selectivity and mediocre activity. Multiple oxidative treatments have shown improvements in the performance of copper catalysts. However, the fundamental underpinning for such enhancement remains controversial. Here, we combine reactivity, in-situ surface-enhanced Raman spectroscopy, and computational investigations to demonstrate that the presence of surface hydroxyl species by co-electrolysis of CO 2 with low concentrations of O 2 can dramatically enhance the activity of copper catalyzed CO 2 electroreduction. Our results indicate that co-electrolysis of CO 2 with an oxidant is a promising strategy to introduce catalytically active species in electrocatalysis. Among all electrocatalysts explored to date, copper (Cu) exhibits the unique capability in reducing CO 2 to valuable hydrocarbons and oxygenates. However, significant enhancement in the rate and selectivity for valuable products and in energy efficiency for Cu-based electrocatalysis remains imperative for this strategy to become industrially viable [1] , [2] , [3] . Oxidative treatments of polycrystalline Cu surfaces have been shown to improve the activity and selectivity towards the production of value-added hydrocarbons and oxygenates, for example, thermal oxidation followed by reduction (so called oxide-derived Cu) [4] , [5] , oxygen plasma activation [6] , and anodic oxidation [7] , [8] , [9] . Although there is a general recognition of the beneficial effect of oxidative treatments on Cu-based catalysts in the CO 2 reduction reaction (CO 2 RR), the mechanisms through which the enhancement is realized remain a topic of considerable discussion. A key point of debate is whether oxygen-containing species, e.g., CuO x , CuO x (OH) y , and Cu(OH) x , are present at the CO 2 RR conditions [6] , [7] , [10] , [11] , [12] , [13] , [14] , [15] , [16] , [17] , [18] , [19] . Multiple ex situ and in situ/operando characterizations lead to contradicting conclusions [6] , [7] , [10] , [11] , [12] , [13] , [14] , [15] , [16] , [17] , [19] . As ex situ measurements have the potential of exposing the sample to the ambient condition, the origin of the oxygen-containing species on the Cu surface detected by these methods is uncertain. Another challenge in resolving this debate is the interfacial sensitivity. As the Pourbaix diagram of Cu shows that only metallic Cu should be present at the reducing environment of the CO 2 RR [20] , the Cu oxide and/or hydroxide species are expected to be present only at the electrode/electrolyte interface, if at all. Thus, the detection of these oxidized Cu species hinges upon the interfacial sensitivity of characterization methods. In this regard, recent in situ/operando surface-enhanced Raman spectroscopic investigations provided initial evidence of the existence of oxidized Cu species at reducing potentials [21] . A much less discussed, but arguably more important, aspect is whether the oxidized Cu species, if they indeed exist at the CO 2 RR conditions, contribute to enhanced reactivity of Cu-based catalysts after oxidative treatments. It is conceivable that Cu oxide and/or hydroxide species are mere spectators during the CO 2 RR, while preferentially exposed facets or defects, e.g., located at the grain boundaries on the metallic Cu surface, induced by the treatment are the real cause of change in the catalytic performance [22] , [23] , [24] , [25] . This has been shown in our recent work in the CO-reduction reaction on Cu [26] . Thus, establishing a direct correlation between the surface speciation of Cu at reaction conditions and reactivity is a frontier in the CO 2 RR research. In this work, we demonstrate that the production rate of oxygenates and hydrocarbons in the CO 2 RR is enhanced by up to 216-fold when coupled with the oxygen reduction reaction (ORR) by co-feeding CO 2 and O 2 (up to 20%). In situ surface-enhanced Raman spectroscopy (SERS) shows that surface hydroxide species on micron-sized Cu particles are present at the CO 2 RR condition, which are likely formed by ORR. The correlation between the surface hydroxyl species and the enhanced reactivity is supported by additional experimental and computational evidence. The addition of low concentrations of H 2 O 2 , a known possible product of the ORR, in the electrolyte results in much less enhancement of catalytic performance as compared to the case of co-reduction of CO 2 and O 2 . Importantly, the Raman feature of the surface hydroxyl group is absent, indicating that the presence of the surface hydroxyl group, rather than any oxidant such as H 2 O 2 , is central to the enhanced production rates. In addition, density functional theory (DFT) calculations show the beneficial role of the surface hydroxyl group in reducing the energy barriers in the formation of oxygenates and hydrocarbons. Results reported in this work demonstrate the promise of enhancing the CO 2 RR performance by leveraging coupled reactions via co-electrolysis. From a practical perspective, the strategy of coupling the CO 2 RR and the ORR could reduce the separation cost of trace amounts of O 2 present in the CO 2 stream from the flue gas or direct air capture. Co-reduction of CO 2 with O 2 The electrolysis experiments are conducted in an H-type electrochemical cell with a standard three-electrode setup (Supplementary Fig. 1 ). Cu electrodes are prepared by depositing commercial polycrystalline Cu powders (~1 μm) (Supplementary Fig. 2 ) onto a PTFE-treated carbon fiber paper. Compared to planar polycrystalline Cu foil electrodes, these electrodes can effectively improve the mass transport of dissolved gas molecules in H-cell configuration [27] , [28] , [29] . To establish the baseline for the co-reduction studies, the CO 2 RR with pure CO 2 is conducted in 0.1 M KHCO 3 (Supplementary Fig. 3a ), and the results are consistent with the previous reports on polycrystalline Cu catalysts [29] , [30] . The major C 2+ products are ethylene, ethanol, n -propanol, and acetate, and the major C 1 products are methane, CO, and formate. The co-electrolysis is performed by feeding a mixture of CO 2 and O 2 with mole ratios of 9:1 and 8:2. The corresponding partial current densities ( j partial ) of C 2+ products, C 1 products and H 2 are color-coded in Figs. 1 and 2 . Fig. 1: Comparison of C 2+ product formations. The partial current densities of C 2+ products measured at 100% CO 2 , 10% O 2 + 90% CO 2 , and 20% O 2 + 80% CO 2 are compared at different potentials of a −0.75 V RHE , b −0.80 V RHE , c −0.85 V RHE , d −0.90 V RHE , e −0.95 V RHE , and f −1.0 V RHE . The numbers stand for the enhancement relative to the rates at pure CO 2 . The error bars represent the standard deviation from at least three independent measurements. Full size image Fig. 2: Comparison of C 1 product and H 2 formations. The partial current densities of C 1 products and H 2 measured at 100% CO 2 , 10% O 2 + 90% CO 2 , and 20% O 2 + 80% CO 2 are compared at different potentials of a −0.75 V RHE , b −0.80 V RHE , c −0.85 V RHE , d −0.90 V RHE , e −0.95 V RHE , and f −1.0 V RHE . The numbers stand for the enhancement relative to the rates at pure CO 2 . The error bars represent the standard deviation from at least three independent measurements. Full size image Remarkably, all C 2+ product formation rates are significantly enhanced in the presence of O 2 in the gas stream (Fig. 1 ). At −0.75 V RHE (Fig. 1a ), the production rate of ethylene, ethanol and acetate shows a more than 20-fold increase with 10% O 2 in the feed. With 20% O 2 , the enhancement for ethylene, ethanol and acetate exceeds 170-fold, 55-fold, and 35-fold, respectively. The formation of n -propanol is also observed at −0.75 V RHE with a partial current density of ~0.5 mA cm − 2 in the presence of O 2 , while no detectable amount of n -propanol is observed at this potential in the oxygen-free atmosphere. The onset potential of n -propanol in the oxygen-free atmosphere occurs at as negative as −0.90 V RHE (Fig. 1d ), and to achieve a similar rate of ~0.5 mA cm − 2 requires an additional 250 mV overpotential, i.e., −1.00 V RHE (Fig. 1f ). Unlike C 2 products, the formation rate of n -propanol does not show a drastic further enhancement as the O 2 ratio increases from 10 to 20%, suggesting its distinct chemistry in forming an additional carbon bond after their common rate-determining step of C–C coupling between two adsorbed CO molecules [29] , [31] , [32] . The oxygen induced enhancement of all C 2+ products is more pronounced at −0.80 V RHE (Fig. 1b ), with higher than 200-fold, 100-fold, and 70-fold increases for ethylene, ethanol and acetate, respectively. As the potential becomes more negative (Fig. 1c–f ), these enhancements start to reduce. At −1.0 V RHE , the increases of C 2+ product formation rates become less than ten times at 20% O 2 . This could be attributed to the enhanced ORR kinetics at higher overpotentials reducing the surface coverage of its intermediates that facilitate the C–C coupling chemistry in the CO 2 RR, as well as the reduced local CO 2 concentration caused by the increased proton consumption rate [33] , [34] . These mechanistic aspects will be discussed in the following sections. C 1 product formation rates in the CO 2 RR are also enhanced in the presence of O 2 (Fig. 2 ). The onset of methane production is improved to as early as −0.75 V RHE in an oxygen-containing atmosphere (Fig. 2a ), while in the absence of O 2 , it is not observed until a much more negative potential of −0.95 V RHE (Fig. 2d ). We emphasize that an increase in the onset potential of at least 200 mV for methane formation with oxygen indicates significantly accelerated reaction kinetics, because an increase in overpotential on this scale could lead to a significant rise in reaction rates (depending on the Tafel slope) assuming the reaction is kinetically controlled near the onset potential. At −0.75 V RHE , the CO formation shows a slightly greater than 5-fold increase and the formate formation shows an approximately two to three times increase with 10–20% oxygen in the reaction atmosphere (Fig. 2a ). As the electrode potential becomes more negatively biased (Fig. 2b–f ), the O 2 induced enhancement in C 1 product formation rates becomes increasingly marginal and turns negative for CO and formate at −0.90 V RHE and below. This trend is more pronounced at the higher (20%) O 2 concentration. The competing hydrogen evolution reaction (HER) is also improved in the presence of O 2 (Fig. 2 ), however, its degree of enhancement is not as sensitive to the applied potential. It should be noted that such significant enhancement for CO 2 RR is not observed on Cu foil electrodes with the addition of 20% O 2 (Supplementary Figs. 4 – 6 ). This could be due to the low solubility of O 2 in the aqueous electrolyte compared with CO 2 (by a factor of ~26) [35] , resulting in the sluggish mass transport of O 2 to the planer electrode surface, and thus diminishing the impact of the ORR on promoting the CO 2 RR. In situ surface-enhanced Raman measurements To understand the mechanism through which co-electrolysis of CO 2 and O 2 boosts the CO 2 RR activity, in situ SERS is employed to identify surface species presenting during the co-electrolysis [36] . The Cu microparticle catalysts employed in this work readily exhibit the surface enhancement of Raman signals, which alleviate the need to introduce SERS-inducing particles [37] , [38] , and is consistent with several recent studies [36] , [37] , [39] . In the Ar atmosphere (Fig. 3a ), multiple peaks at 146, 219, 412, 528, and 619 cm −1 are observed at the open circuit potential (OCP) and can be attributed to the surface Cu 2 O (Cu 2 O surf ) [21] , [40] . These peaks decrease in intensity as the potential becomes more negative and disappear at 0 V RHE , due to the reduction of Cu 2 O surf , and no other peak is observed at more negative potentials. An additional band at 360 cm −1 appears after the removal of Cu 2 O surf at 0 V RHE in the CO 2 atmosphere (Fig. 3b ), whose assignment remains debated in the literature [36] , [41] , This band disappears at −0.4 V RHE , likely due to the conversion of adsorbed CO to other products at more negative potentials, and thus the corresponding species is unlikely to have a major impact on the CO 2 RR. A prominent band at 706 cm −1 appears at potentials below 0 V RHE in the O 2 atmosphere (Fig. 3c ), which has been assigned to the surface hydroxyl species [21] . Control experiment in D 2 O shows a redshift of this band to 668 cm −1 (Fig. 3c ), which confirms the binding of a protonated atom. Although the isotopic shift when switching from H 2 O to D 2 O is larger than that estimated based on the reduced mass of a [Cu-]O-H(D) bending mode (~20 cm −1 ), this is likely due to the presence of solvent. It is reasonable to assume that there is substantial hydrogen bonding between Cu-OH and the H in the surrounding water molecules, which will impact on the frequency of the Cu-OH mode. When replacing H 2 O with D 2 O, we not only replace Cu-OH with Cu-OD, but also replacing the surrounding H 2 O with D 2 O, thus the change in the reduced mass is expected to be more significant than that without the hydrogen-bonded water. The possibility of this band at 706 cm −1 corresponding to an adsorbed C-containing species is ruled out by the observation that this band only appear in O 2 contained electrolyte but not in pure CO 2 or Ar saturated electrolyte (Fig. 3 ). Electrolysis using 13 CO 2 is helpful to further confirm this argument. However, we believe the current evidences are sufficient to support the assignment of the 706 cm −1 band to surface hydroxyl, rather than a C-containing species. Surface hydroxyl species in the O 2 atmosphere is likely formed during the 4-electron pathway in the conversion of O 2 to H 2 O (Supplementary Fig. 7 ), as it is a known intermediate in the ORR on multiple metal surfaces [42] . Interestingly, the Cu 2 O surf appears to persist to lower potentials in the O 2 atmosphere as the broad peak at 430–650 cm −1 corresponding to Cu 2 O surf does not completely disappear until −0.5 V RHE [21] , [36] . In the atmosphere of 10% O 2 + 90% CO 2 , the SER spectra exhibit features of those from in both O 2 and CO 2 atmospheres (Fig. 3d ). Importantly, the key difference between the SER spectra in the CO 2 and O 2 + CO 2 atmospheres is the presence of the band corresponding to the surface hydroxyl species. This is an indication that the presence of the surface hydroxyl group, corresponding to a Raman band at 706 cm −1 , is responsible for the distinct reactivities in the CO 2 RR in the absence and presence of O 2 in the reaction atmosphere (Fig. 3e ). SER spectra with extended spectral windows are included in the Supplementary Figs. 8 and 9 and the related peaks are discussed in Supplementary Note 1 . Fig. 3: In situ surface-enhanced Raman spectroscopy. Raman spectra of Cu catalyst at electrolysis with a pure Ar gas feed in 0.1 M KHCO 3 /H 2 O; b pure CO 2 gas feed in 0.1 M KHCO 3 /H 2 O; c pure O 2 gas feed in 0.1 M KHCO 3 /H 2 O and 0.1 M KDCO 3 /D 2 O; d 10% O 2 + 90% CO 2 in 0.1 M KHCO 3 /H 2 O. e Schematic of CO 2 RR on Cu surface at the presence of hydroxyl groups induced by ORR. Full size image The CO 2 RR activity and spectroscopic results show that the formation of H 2 O 2 is unlikely the cause of the enhanced CO 2 RR performance during the co-electrolysis with O 2 . H 2 O 2 is a possible product of the ORR via the 2-electron pathway [43] . If produced during the co-electrolysis of CO 2 and O 2 on Cu, H 2 O 2 could potentially modify the surface speciation and impact of the rate and product distribution of the CO 2 RR. Introducing up to 10 mM of H 2 O 2 in the electrolyte of the CO 2 RR (with a pure CO 2 feed) leads to a relatively modest change, i.e., less than 10-fold increase, in the production rates of oxygenates and hydrocarbons (Supplementary Fig. 10 ), which is in stark contrast with the observation of co-electrolysis with O 2 (Figs. 1 b and 2b ). This is consistent with the observation that the ORR occurs mainly through the 4-electron pathway on the Cu surface (Supplementary Fig. 7 ) and thus the production of H 2 O 2 is expected to be negligible. Furthermore, in situ SER spectra using electrolyte (CO 2 saturated 0.1 M KHCO 3 ) with up to 10 mM of H 2 O 2 do not show any detectable feature corresponding to the hydroxyl species (Supplementary Fig. 11 ), suggesting distinct reduction mechanisms and intermediates in the ORR and the H 2 O 2 reduction on Cu. As the H 2 O 2 concentration in the electrolyte increases, the Raman features corresponding to Cu 2 O surf persists to more negative potentials (Supplementary Fig. 11 ), which is expected as H 2 O 2 is a potent oxidant. Importantly, the lack of the surface hydroxyl group and the modest change in the CO 2 RR activity with added H 2 O 2 support the hypothesis that the surface hydroxyl group formed during the co-electrolysis is responsible for the enhanced CO 2 RR performance. Density functional theory calculations To further evaluate the hypothesized beneficial effect of the hydroxyl group on the CO 2 RR, potential energy landscapes of key reaction steps are estimated via density functional theory calculations. The free energy profiles of the rate-determining steps (RDS) in the formation of C 2+ products, i.e., *CO dimerization [29] , [31] , [44] , [45] and methane, i.e., *CO hydrogenation [29] , [44] , [46] , are calculated at different *OH coverage on the Cu(100) facet, with the representative model structures and results shown in Figs. 4 and 5 , respectively [31] , [45] , [46] . −0.5 V SHE (i.e., equivalent to −0.9 V RHE ) is chosen as the potential in our calculations. Cu(100) facet is employed for the computational study. Cu(100) and Cu(111) are the most exposed facets on polycrystalline Cu surface because of their low surface energies [47] . It has been shown that polycrystalline Cu surface undergoes surface reconstruction to form Cu(100) under the CO 2 RR conditions, which is also consistent with experiments showing that polycrystalline Cu leads to a product distribution similar to that on Cu(100) [48] . Therefore, Cu(100) facet is commonly used as a representative model surface for obtaining theoretical insights into experimental studies based on polycrystalline Cu [46] , [49] . Our computational model also consists hollow-site adsorbed *OH with different coverage. This is because *OH is most stable on hollow sites at the negative potentials described by the VASPsol model. The vibrational modes for hollow-site *OH in the vicinity of *CO were calculated at the initial states of *CO dimerization and *CO hydrogenation (Supplementary Tables 1 and 2 ). We employ a well-established finite difference method to calculate the vibrational modes of the *OH adsorbate [49] , [50] . The calculated wavenumbers of vibration modes of *OH are compared with the Raman band observed experimentally. The results show good agreement with the observed Raman band of 706 cm −1 in the in situ SERS experiments, which supports the representativeness of the computational model employed in this work. Due to the limitations of DFT calculations, other characters such as band width and intensity, cannot be accurately predicted and thus are not discussed. Fig. 4: Computational model. Representative structures of *CO dimerization at initial states ( a ), transition states ( b ), and final states ( c ). Representative structures of *CO hydrogenation at initial states ( d ), transition states ( e ), and final states ( f ). Full size image Fig. 5: Free energy diagram. a *CO dimerization. b *CO hydrogenation. The binding free energies for initial states and transition states at different *OH coverage are calculated with reference to a Cu slab with specific numbers of *OH, gas phase CO, H 2 , and liquid H 2 O molecules. The potential is −0.5 V SHE (i.e., equivalent to −0.9 V RHE ). ΔΔ G (ΔΔ G ≠ ) is defined as the reaction-free energy (free energy barrier) at certain *OH coverage referenced to the value obtained at zero *OH coverage (see “Methods” section for computational details). Full size image Both the activation barrier and the free energy change for *CO dimerization decrease as the *OH coverage increases from 0 to 3/9 but rebound with further increase in *OH coverage (Fig. 5a ). Both the initial state and transition state become less stable as the *OH coverage increases. This could be attributed to the increase of oxidation state of surface Cu as revealed by Bader charge analysis (Supplementary Fig. 12 ), which weakens the π-back-donation from the Cu to the anti-bonding orbital of the C≡O bond [51] , [52] . The magnitude of destabilization of the initial state is greater than that of the transition state when the *OH coverage is at or below 3/9, leading to the decrease of the reaction barrier. This is consistent with the observed enhancement of C 2+ product formation rate with ≤20% O 2 in the gas feed (Fig. 1 ). As the *OH coverage increases beyond 3/9, both the activation barrier and the free energy change for *CO dimerization increase substantially, which is likely due to the repulsive interaction with the excess *OH groups nearby. For *CO hydrogenation to *CHO, both activation barrier and free energy change decrease substantially when *OH coverage increases from 1/9 to 4/9 (Fig. 5b ). Notably, these decreases are much more significant than those in *CO dimerization, which agrees with the significant anodic shift of methane onset potential in the presence of the concurrent ORR (Fig. 2 ). The energies of initial structures fluctuate slightly within an energy range of 0.2 eV when *OH coverage increases, however, the transition state of *CO hydrogenation is stabilized under same conditions. We speculate that this is likely due to the transition state forms additional hydrogen bonds with *OH groups at higher coverage. The stabilization of reactant by forming hydrogen bonds with *OH has been reported in a previous work [53] . A key difficulty in elucidating the role of oxidized Cu species on the surface in promoting the CO 2 RR is their poor stability under the reducing condition, which renders their composition and structure ambiguous. This stems from the fact that these species are prepared at a more oxidizing atmosphere, thermochemically or electrochemically, and then brought to a reducing environment. This challenge is circumvented by providing a continuous supply of oxidant in the CO 2 RR, i.e., co-electrocatalysis of CO 2 and O 2 , to stabilize the surface oxidized Cu species, i.e., surface hydroxyl group. Co-electrolysis could also be viewed as coupled reactions, with the ORR supplying reactive oxygen species to form and replenish the surface hydroxyl species vital to the enhancement of the CO 2 RR. Control experiments with H 2 O 2 show that it is not H 2 O 2 or intermediates of its reduction because neither the CO 2 RR activity nor the spectral feature with H 2 O 2 resembles that in the co-electrolysis at otherwise identical conditions. The presence of H 2 O 2 in the electrolyte makes Cu 2 O surf more resistant to negative potentials (Supplementary Fig. 11 ), even to −0.8 V RHE at 10 mM of H 2 O 2 . The fact that H 2 O 2 does not significantly promote the CO 2 RR shows that the CO 2 RR performance is highly sensitive to the nature of the surface species. As different oxidants lead to different surface species, results reported in this work establish a paradigm for enhancing the CO 2 RR by co-electrolyzing CO 2 with an oxidant. The nature and concentration of oxidants could be designed to tune the nature and coverage of surface oxidized Cu species. This hypothesis is supported by the contrasting results of using H 2 O 2 and O 2 oxidant, as well as different partial pressure of O 2 . Higher partial pressure of O 2 in the feed (up to 20%) is expected to increase the surface coverage of the adsorbed hydroxyl species, which is generally beneficial toward the improvement of production rates of oxygenates and hydrocarbons. The diminishing impact of O 2 on the CO 2 RR at potentials below −0.9 V RHE could be attributed to at least two factors: (1) Reduction of surface coverage of the hydroxyl species due to its facile reduction at such negative potentials; unfortunately, excessive bubble formation prevents spectroscopic investigations at these potentials. (2) Reduction in the local CO 2 concentration due to the accelerated CO 2 RR and increased alkalinity caused by the fast proton consumption from both the CO 2 RR and the HER [33] , [34] . The increase of electrolyte pH has been demonstrated to not affect C 2+ product formations because the RDS does not involve any proton transfer [28] , [44] , [54] , [55] . However, higher pH is known to increase the hydrogen binding energy (HBE) [56] , [57] , which accelerates the HER on Cu [58] . This is consistent with the observed enhancement in the HER rate with the addition of O 2 (Fig. 2 ). The enhancement of HER rate is relatively insensitive to the applied potential. This is likely due to the interfacial pH at the cathode does not change significantly with electrolysis potentials because the ORR is severely mass-transport limited at such large overpotentials (>1.8 V). In addition to enhancing the CO 2 RR rates, the introduction of O 2 also significantly reduces the Faradaic efficiency (FE) of CO 2 RR products (Supplementary Fig. 3b, c ), presumably by introducing a competing reaction, i.e., the ORR. We note that at higher O 2 concentrations than 20%, a limited increase in the production rate of the CO 2 RR with elevated ORR activity and reduced Faradaic efficiency for the CO 2 RR are expected based on current results. Reliable measurements of electrolysis at higher O 2 concentrations are challenging due to the instability of the electrode at high current densities (over 100 mA cm − 2 ) in an H-type electrochemical cell. Systematic investigations of the impact of O 2 partial pressure on the CO 2 RR activity require enhanced mass transport which could be more easily accomplished in flow cell configurations [59] , [60] , [61] , [62] , and are outside the scope of this proof-of-concept work. It is important to note that any practical CO 2 source contains large quantities of O 2 can be utilized, e.g., flue gas from power plants or air, so CO 2 RR systems that are tolerant to or enhanced by a low concentration of O 2 in the feed could significantly reduce the separation cost. In the meantime, co-electrolysis of other oxidants, e.g., peroxyacetic acid, ammonium persulfate, could be a fruitful strategy to further improve the rate and efficiency of CO 2 RR. Materials The polycrystalline Cu powder (−625 mesh, APS 0.50–1.5 micron, 99% metal basis) is purchased from Alfa Aesar. Cu foil (0.1 mm thick, 99.9999% metal basis) is purchased from Alfa Aesar. Potassium carbonate (99.997% trace metals basis) is purchased from Alfa Aesar. Chelex 100 sodium form is purchased from Sigma-Aldrich. Isopropanol (99.999% trace metal basis) is purchased from Sigma-Aldrich. Dimethyl sulfoxide (≥99.9%) is purchased from Alfa Aesar. Deuterium oxide (99.9 atom% D) is purchased from Sigma-Aldrich. Nafion solution (5 wt%) is purchased from Sigma-Aldrich. Phosphoric acid (ACS reagent, ≥85 wt% in H 2 O) is purchased from Sigma-Aldrich. Graphite rod (99.995% trace metals basis) is purchased from Sigma-Aldrich. Sigracet 39 BC carbon fiber paper is purchased from Fuel Cell Store. Carbon Dioxide (99.999%), oxygen (99.999%), and argon (99.999%) are purchased from Air Liquide. All electrolyte solutions are prepared using Milli-Q water (18.2 MΩ cm). Electrode preparation To prepare the polycrystalline Cu power electrode, an ink solution is first prepared by mixing 1 mg Cu powder and 1 mL isopropanol followed by sonicating for 20 min. 900 μL of ink solution is dropcasted onto the microporous layer of a 3 × 3 cm 2 Sigracet 39 BC carbon fiber paper. After drying in air, 180 μL of 2.5 wt% Nafion solution (diluted with isopropanol) is uniformly deposited onto the catalyst surface. The catalyst is dried in the air again and transferred into a vacuum box to thoroughly remove the residual solvent. The catalyst is then cut into small pieces with a size of 0.6 × 1.5 cm 2 and a nickel wire current collector is attached to a piece of the catalyst using silver epoxy. To prepare the electropolished Cu foil electrode, a nickel wire current collector is welded to a piece of Cu foil. The electrode is then electropolished in 85% phosphoric acid at 2.1 V versus a graphite rod electrode for 5 min followed by rinsing with Mill-Q water (18.2 MΩ cm). A fresh working electrode is used for each electrochemical measurement. Electrochemical measurements All electrochemical measurements are conducted in a custom designed gastight two-compartment electrochemical cell fabricated by Adams & Chittenden Scientific Glass with three-electrode configuration. A graphite rod is used as counter electrode and a Ag/AgCl (3.0 M, BASi) electrode is used as reference electrode. The two chambers of the electrochemical cell are separated by anion-exchange membrane (Selemion AMV, AGC Inc.). The electrolyte used for all electrochemical measurements is CO 2 -saturated 0.1 M KHCO 3 solution with a pH of 6.8, which is prepared by purging 0.05 M K 2 CO 3 solution with CO 2 overnight, and the electrolyte is purified with Chelex before electrolysis. All electrochemical measurements are conducted using a Gamry Reference 600+ Potentiostat and the measured potential is converted to RHE scale using the following formula: E RHE = E Ag/AgCl + 0.210 + 0.05916 × pH (in volts), where the standard value for the Ag/AgCl reference electrode is calibrated using a homemade standard hydrogen electrode. The uncompensated resistance ( R u ) is measured by potentiostatic electrochemical impedance spectroscopy and 100% of R u is compensated by the potentiostat during electrolysis. All electrodes are pretreated in Ar-purged electrolyte at −1 V RHE for 5 min to stabilize surface conditions. The gas flow is then switched to reactant gas (pure CO 2 or 10% O 2 + 90% CO 2 or 20% O 2 + 80% CO 2 ) and the system is purged for 15 min prior to a 1 h electrolysis. All gases are directly delivered into electrolyte through a gas dispersion frit at a total flow rate of 10 mL/min. The flow rate is controlled by mass flow controllers (MKS Instruments Inc.) and calibrated by an ADM flow meter (Agilent Technologies). The O 2 + CO 2 mixture is prepared by mixing CO 2 and O 2 at desired ratio using mass flow controllers at a total flow rate of 10 mL/min. The outlet flow of the electrochemical cell is directly vented to the sample loop of a gas chromatograph (Agilent 7890B) for product quantification. Product quantification The gaseous products are quantified every 20 min using a gas chromatograph (GC) (Agilent 7890B) equipped with a ShinCarbon ST column and a HayeSep Q column. A thermal conductivity detector is used to quantify H 2 and a flame ionization detector with a methanizer is used to quantify CO, CH 4 , and C 2 H 4 . Ar is used as carrier gas. The analysis results of three GC analyses during the 1 h electrolysis are averaged. The liquid products are quantified using 1 H NMR on a Bruker AVIII 400 MHz NMR spectrometer after the whole electrolysis process. The NMR sample is prepared by mixing 500 μL of the electrolyte collected after electrolysis with 100 μL of internal standard solution (1.67 ppm (m/m) dimethyl sulfoxide in D 2 O). The water signal is suppressed using the presaturation method. Determination of ORR electron transfer number The ORR electron transfer number of polycrystalline Cu powder catalyst is determined using rotating disk electrode (RDE) measurement and Koutecký–Levich equation method. To prepare the electrode for RDE measurement, an ink solution is first prepared by mixing 5 mg Cu powder, 25 μL Nafion solution and 1 mL 2-propanol followed by sonicating for 30 min in an ice cold water bath. A 20 μL ink is then dropcasted onto a glassy carbon rotating disk electrode (0.5 cm diameter, Gamry). A graphite rod is used as counter electrode and a double junction Ag/AgCl electrode (3.0 M) is used as reference electrode. The experiments are conducted using a Gamry RDE 710 system and the electrolyte is 0.1 M KHCO 3 solution. The cyclic voltammogram (CV) is firstly taken under Ar at a scan rate of 10 mV/s with a rotation speed of 2500 rpm prior to ORR measurement. The electrolyte is then bubbled with O 2 for at least 20 min to saturate the electrolyte. CVs in O 2 atmosphere are recorded at various rotation speed (400, 625, 900, 1225, 1600, 2025, and 2500 rpm) at a scan rate of 10 mV/s. In situ Raman spectroscopy measurements In situ Raman spectroscopy measurements are conducted using a custom-made three-electrode electrochemical cell in H-cell configuration that consists two compartments and is separated by a piece of Nafion ion exchange membrane (IEM, Nafion 211, Fuel Cell Store) (Supplementary Fig. 13 ). The three-electrode system is made up of a Cu working electrode that is identical to the ones in reactivity measurement, a Ag/AgCl reference electrode (3.0 M NaCl, BASi) and a graphite counter electrode. A potentiostat (VersaSTAT, Princeton) is used to perform electrolysis. Electrolyte saturated with desired gas is delivered into the cell using a HPLC pump (GP50 Gradient Pump, Dionex) to achieve similar mass transport as in magnetically stirred reactivity cell. The Raman spectroscopy measurements are carried out using LabRAM HR Evolution microscope (Horiba Jobin Yvon) equipped with a 632.8 nm He-Ne laser, a ×50 objective (NA = 0.55), and a CCD detector. The filter is set to be 50% to keep a low laser intensity to avoid any irradiation-induced modifications of Cu surface. The acquisition time is 20 s for each spectrum with the accumulation times of 2. Computational details The Cu(100) metal slab (3 × 3) consisting of three layers with the bottom layer fixed in its bulk position is employed to simulate the surface of Cu. The total energy of the slab with different adsorbates are calculated using DFT with the Perdew–Burke–Ernzerhof exchange-correlation functional in plane-wave pseudopotentials, as implemented in the Vienna ab initio Simulation Package (VASP) [63] . The empirical D2 approach as implemented in VASP is employed to describe the van der Waals interactions. All calculated energy values are extrapolated to k B T = 0. A Monkhorst–Pack k-point net of 3 × 3 × 1 is chosen to sample the reciprocal space. A vacuum of 25 Å is introduced to each side to avoid interactions between successive metal slabs. VASPsol model is employed to establish the electrochemical interface [64] , [65] . In this model, the Fermi energy is adjusted to a target value by changing the number of electrons in the system during each step of the geometry optimization, which keeps the work function and electrode potential constant in the calculations. Then the linear Poisson–Boltzmann implicit solvation model with a Debye screening length of 3.0 Å is used to neutralize the non-zero charge in the simulation cell and simulate water and the electrolyte, allowing for a more realistic description of the electrochemical double layer. A detailed description of this approach has been provided in our previous work [66] , [67] , [68] . The transition state for each reaction is first approached using the nudged elastic band (NEB) method in the neutral state. Forces on the climbing image are converged to <0.02 eV/Å. The plane-wave cutoff, smearing parameter and functional, and calculator parameters are the same as those used in slab geometry optimizations. Structures obtained from NEB are employed to generate the input structure and orientation for the dimer calculation. The force of the dimer calculation is converged to <0.1 eV/Å to accurately locate the saddle point, i.e., the transition state. After that, the free energy of transition state is calculated under constant potential. In the calculations for *CO hydrogenation, the required H + / e − pair for reduction is assumed to originate from the aqueous solution and the electrode. Its free energy is estimated based on the computational hydrogen electrode model [69] . In addition to the implicit Poisson–Boltzmann solvation model, all the stationary points along the hydrogenation step are solvated by four explicit water molecules to provide a better description of the solvent. All possible structures, including different adsorption sites of *CO and *OH, relative position between *CO and *OH, etc., are investigated at all *OH coverage. The most stable structures are employed to investigate the impact of *OH adsorbate to the RDS of C 2+ product formations and CH 4 formation (Supplementary Figs. 14 – 17 ). The free energies of the slab systems were calculated as follows: 
    G = E_elec^solv + ZPVE + H_vib - TS_vib,
 (1) where \(E_{{\mathrm{elec}}}^{{\mathrm{solv}}}\) was the electronic energy of the system calculated from VASPsol. We treated all degrees of freedom of the adsorbates as vibrational and neglect the contribution of vibrations of the slab. The vibrational frequencies ( ν ) were evaluated by calculating the partial Hessian matrix through the finite difference method. Unusually low vibrational modes (<50 cm −1 ) were reset to 50 cm −1 to avoid unphysically large entropy contributions. Based on the calculated vibrational frequencies, we calculated the zero-point vibrational energy (ZPVE), vibrational contributions to the internal energy ( H vib ) and entropy ( S vib ) at 298 K as follows: 
    ZPVE = ∑_νhν/2,
 (2) 
    H_vib = ∑_νhν/e^hν /k_BT - 1,
 (3) 
    S_vib = k_B∑_ν[ hν/k_BT( e^hν /k_BT - 1) - ln( 1 - e^ - hν /k_BT)]. (4) The free energies of the molecules were determined as follows: 
    G = E_elec^solv + ZPVE + ( n/2 + 1)k_BT + H_vib - T(S_vib + S_trans + S_rot),
 (5) where n is 6 for non-linear molecules and 5 for linear molecules. ZPVE was calculated as shown above. H vib , S vib , S rot , and S trans were obtained from Jaguar using the PBE/6-31G* basis set. 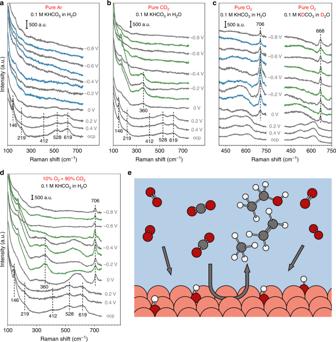Fig. 3: In situ surface-enhanced Raman spectroscopy. Raman spectra of Cu catalyst at electrolysis withapure Ar gas feed in 0.1 M KHCO3/H2O;bpure CO2gas feed in 0.1 M KHCO3/H2O;cpure O2gas feed in 0.1 M KHCO3/H2O and 0.1 M KDCO3/D2O;d10% O2+ 90% CO2in 0.1 M KHCO3/H2O.eSchematic of CO2RR on Cu surface at the presence of hydroxyl groups induced by ORR. The correction terms of all free energies are provided in Supplementary Table 3 . 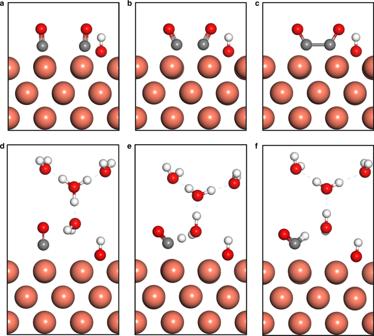Fig. 4: Computational model. Representative structures of *CO dimerization at initial states (a), transition states (b), and final states (c). Representative structures of *CO hydrogenation at initial states (d), transition states (e), and final states (f). 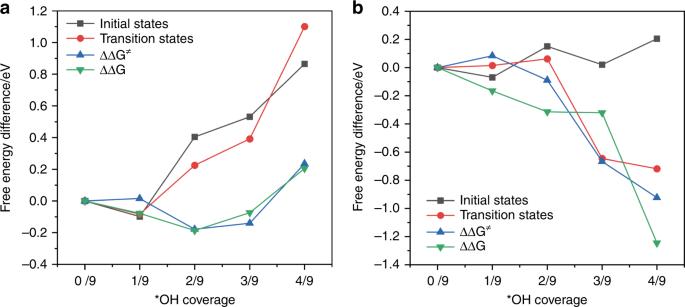Fig. 5: Free energy diagram. a*CO dimerization.b*CO hydrogenation. The binding free energies for initial states and transition states at different *OH coverage are calculated with reference to a Cu slab with specific numbers of *OH, gas phase CO, H2, and liquid H2O molecules. The potential is −0.5 VSHE(i.e., equivalent to −0.9 VRHE). ΔΔG(ΔΔG≠) is defined as the reaction-free energy (free energy barrier) at certain *OH coverage referenced to the value obtained at zero *OH coverage (see “Methods” section for computational details). For *CO dimerization, the adsorption free energy of each state was calculated as: 
    G_abs^IS( n/9 ^∗OH coverage) = G_IS( n/9 ^∗OH coverage) - G_Cu + n^∗OH-2G_^∗CO,
 (6) 
    G_abs^TS( n/9 ^∗OH coverage) = G_TS( n/9 ^∗OH coverage) - G_Cu + n^∗OH-2G_^∗CO,
 (7) 
    G_abs^FS( n/9 ^∗OH coverage) = G_FS( n/9 ^∗OH coverage) - G_Cu + n^∗OH-2G_^∗CO. (8) For *CO hydrogenation, the adsorption free energy of each state was calculated as: 
    G_abs^IS( n/9 ^∗OH coverage) = G_IS( n/9 ^∗OH coverage) - G_Cu + n^∗OH-G_^∗CO-4G_H_2O,
 (9) 
    G_abs^TS( n/9 ^∗OH coverage) =   G_TS( n/9 ^∗OH coverage) - G_Cu + n^∗OH
     -  G_^∗CO-4G_H_2O-1/2G_H_2,
 (10) 
    G_abs^FS( n/9 ^∗OH coverage) =   G_FS( n/9 ^∗OH coverage)
     -  G_Cu + n^∗OH-G_^∗CO-4G_H2O-1/2G_H_2. (11) For the results presented in Fig. 5 : 
    ΔG_abs^IS( n/9 ^∗OH coverage) = G_abs^IS( n/9 ^∗OH coverage) - G_abs^IS( zero coverage),
 (12) 
    ΔG_abs^TS( n/9 ^∗OH coverage) = G_abs^TS( n/9 ^∗OH coverage) - G_abs^TS( zero coverage),
 (13) 
    ΔΔG = ΔG( n/9 ^∗OH coverage) - ΔG( zero ^∗OH coverage),
 (14) 
    ΔΔG^  = ΔG^ ( n/9 ^∗OH coverage) - ΔG^ ( zero ^∗OH coverage),
 (15) where 
    ΔG( n/9 ^∗OH coverage) = G_abs^FS( n/9 ^∗OH coverage) - G_abs^IS( n/9 ^∗OH coverage),
 (16) 
    ΔG^ ( n/9 ^∗OH coverage) = G_abs^TS( n/9 ^∗OH coverage) - G_abs^IS( n/9 ^∗OH coverage),
 (17) are the free energy change and free energy barrier for the reaction (*CO dimerization or *CO hydrogenation) at certain *OH coverage, respectively. Physical characterization The microstructure of the Cu catalyst is characterized by field emission scanning electron microscope (Merlin FE-SEM, Zeiss). Powder X-ray diffraction pattern is collected using a Rigaku MiniFlex 600 with Cu Kα radiation. X-ray photoelectron spectroscopy measurements are conducted on a PHI Quantera II and CasaXPS software (Casa Software Ltd., UK) is used to analyze the resulting spectra.